Topological zoo of free-standing knots in confined chiral nematic fluids Knotted fields are an emerging research topic relevant to different areas of physics where topology plays a crucial role. Recent realization of knotted nematic disclinations stabilized by colloidal particles raised a challenge of free-standing knots. Here we demonstrate the creation of free-standing knotted and linked disclination loops in the cholesteric ordering fields, which are confined to spherical droplets with homeotropic surface anchoring. Our approach, using free energy minimization and topological theory, leads to the stabilization of knots via the interplay of the geometric frustration and intrinsic chirality. Selected configurations of the lowest complexity are characterized by knot or link types, disclination lengths and self-linking numbers. When cholesteric pitch becomes short on the confinement scale, the knotted structures change to practically unperturbed cholesteric structures with disclinations expelled close to the surface. The drops with knots could be controlled by optical beams and may be used for photonic elements. The complexity and versatility of knots have fascinated humanity for centuries, and since the pioneering work of Kelvin and Tait [1] , [2] , they have been systematically studied as idealized topological entities [3] . Knotting and linking are not limited to ropes [4] and are observed even at a molecular level in DNA [5] , [6] , polymers [7] , [8] and single molecules [9] . However, the intricacy of knots in physical systems extends beyond basic mathematical notions of knot theory if the knot is a part of a continuum field. The coexistence of the knot and the surrounding physical field leads to additional topological and energetic constraints, stability issues and the problem of precise material manipulation and experiment design, required to create the knots. Recently, knotted field structures have been observed and engineered in optical fields [10] , fluid vortices [11] , quantum states [12] and liquid crystals (LCs) [13] , [14] , [15] . As a medium that allows topologically stable disclinations (defect lines in the nematic order parameter field), nematic LCs are a choice component in composite materials. The first linked disclinations in chiral nematics, albeit transient and non-singular, were observed by Bouligand [16] , [17] . With the aid of optical manipulation, the topological properties of closed disclination loops have been probed more systematically in experiments involving entanglement of colloidal particles. The entanglement enabled creation of robust chains and two-dimensional (2D) colloidal crystals, but also revealed that the disclinations can be formed into knots and links of arbitrary complexity [13] , [14] . Studying knotted disclinations in LCs offers a unique opportunity for probing the most complex aspects of their topological properties. It advances theoretical understanding of the intricate topological nature of the material and drives the improvement of precise experimental techniques needed to control such structures. Variety of the complex metastable structures, combined with fine experimental control thus sets a path to creation of new topologically driven materials. Contrary to the case of nematic colloids [18] , where topology is tuned by imposing complex boundary conditions in an infinitely extending nematic field, nematic droplets offer a different kind of frustration. The closed spherical boundary removes the existence of a preferred axis, restoring the orientational isotropy of the system and removing the influence of far-field imposed by external boundaries. In nematic droplets, the structure is thus influenced primarily by the anchoring condition. The defect behaviour in droplets with the anchoring varying from homoeotropic (molecules aligned normal to the surface) to planar degenerate (molecules parallel to the surface) is well researched both topologically and experimentally [19] , [20] , [21] . In any case, however, the disclinations in an ordinary nematic tend to shorten as much as possible to minimize the costly isotropic cores and the absence of obstructions inside the droplet leads to highly symmetric structures of point defects and ring disclinations. A way around this setback is to use chiral nematic LCs (cholesterics). In cholesterics, the intrinsic chirality causes the director n , denoting the average orientation of the LC molecules, to spontaneously form a helical twist. This twisting can act as an obstruction to kinetically trap disclination lines and prevent the otherwise favourable shortening and merging process. The distance over which the director turns by 2π, known as the intrinsic cholesteric pitch p 0 , can be controlled by temperature [22] , optical illumination [23] or chiral dopants [24] . The periodic modulation of the average orientation effectively changes the optical axis, achieving specific optical characteristics of cholesterics. Introducing chirality to the LC droplets breaks the rotational symmetry of the nematic texture inside the droplet. The tendency to create layer-like helical structure competes with the spherical boundary conditions of the droplet, creating a frustrated environment with a multitude of metastable states [21] , [25] , [26] , [27] . Ensuing conformations not only depend on the anchoring, but vary continuously with the cholesteric pitch. The structures with concentric layers found in cholesteric droplets with degenerate planar anchoring have lately attracted much attention with their use in advanced soft matter photonic elements such as Bragg resonators for micro lasers [28] , [29] , [30] , [31] , [32] . The recent detailed numerical and topological study of these systems shows [27] that the degenerate boundary conditions still allow enough degrees of freedom to at least partially accommodate the requirements of the intrinsic twisting and form rather simple defect structures. Homoeotropic boundary condition, on the other hand, is much more restrictive and induces formation of disclinations even at a flat interface [33] , [34] . In a droplet, the inability of disclinations to pass through the boundary only allows confined closed disclination loops, which motivates our quest for knotted structures. While for a cholesteric with very large pitch (effectively nematic) the ground state with only a few metastable states is well researched, many different metastable states could be expected with shorter pitch. Unlike in the colloidal systems, where entangled disclinations stay close to the surface, the inverted geometry of droplets allows the bulk interior to stabilize the disclinations in three dimensions. For this reason, the homoeotropic cholesteric droplets are an ideal model system for the search of free-standing knotted disclination structures. In this article, we demonstrate the possibility to produce and manipulate metastable free-standing knots and links of topological defect lines by using a simulated thermal quench in the ordering field of spherical cholesteric LC droplets with surfaces inducing strong but finite normal (homoeotropic) orientation of the molecules. We first show that by simulated thermal quench, a variety of metastable configurations (that is, configurations that are local minima of the free energy) can be produced that mainly differ in the type of the knot or link that the topological defect lines tie. We analyse the variety of possible states, with their complexity primarily depending on the intrinsic chirality of the medium, but with chirality sufficiently low that the blue phases are not yet stable. We study the disclination lines and show how the topological constraints are satisfied. Finally, we discuss the difference in the nature of observed structures for droplets with varying degrees of chirality, and the behaviour in the limiting case of cholesterics with a high degree of chirality. Simulated temperature quench When shortening the pitch, one would expect a variety of metastable states due to the competition between cholesteric layered ordering and spherical bounding surface. Experimentally (and also numerically), obtaining the states with higher energy than the ground state can often be challenging. A way to produce the metastable structures, despite the energetic barriers between the states, is to repeatedly relax the LC from a randomly selected disordered state [35] . To experimentally attain such a state, the LC is heated above the nematic-isotropic transition temperature and then left to quickly cool down to room temperature. Numerically, the thermal quench is produced by setting the initial condition of the director to random vectors at each mesh point and then numerically relaxing the system as can be seen in Fig. 1a,b . The numerical quench that we use is very similar to the experimental thermal quench [36] . As we are interested in steady states, our numerical algorithm follows the orientational relaxation but neglects hydrodynamic aspects that would primarily cause the anisotropy in the dynamics of disclinations with different winding numbers [37] , [38] . Details are described in the Methods section. 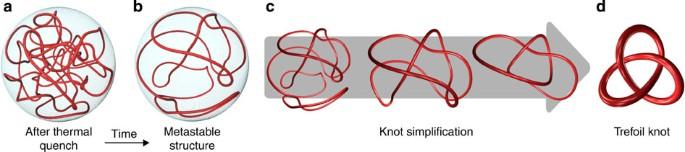Figure 1: Randomly occurring knots in homoeotropic cholesteric droplets. (a) A highly disordered state forN=5 shortly after the numerically simulated thermal quench. Note a ‘zoo’ of disclination lines in red, visualized asS=0.48 isosurfaces of the nematic degree of order. After a few millions of simulation steps the system relaxes to a (b) metastable state as a local free energy minimum. (c) By extracting and geometrically simplifying the disclination line, a knot can be deciphered as a (d) trefoil knot. Figure 1: Randomly occurring knots in homoeotropic cholesteric droplets. ( a ) A highly disordered state for N =5 shortly after the numerically simulated thermal quench. Note a ‘zoo’ of disclination lines in red, visualized as S =0.48 isosurfaces of the nematic degree of order. After a few millions of simulation steps the system relaxes to a ( b ) metastable state as a local free energy minimum. ( c ) By extracting and geometrically simplifying the disclination line, a knot can be deciphered as a ( d ) trefoil knot. Full size image After a thermal quench, domains of local LC order are established, producing a zoo of randomly positioned singular nematic disclination lines with winding number −1/2 between the domain walls, as visualized in Fig. 1a . The relaxation leads to coarsening of the disclination network until the few remaining disclination lines reach an equilibrium with the compression and distortion of the cholesteric helix and thus become kinetically trapped ( Fig. 1b ). The resulting metastable structures often include knotted or linked disclinations. Note that all disclinations in equilibrium droplets are simple singular nematic disclinations with winding number −1/2 but the chirality actually prevents them from minimizing their lengths as typically happens in non-chiral nematics. After numerically extracting the curve of the disclination from the equilibrated numerical sample, we simplify its geometry with dedicated software ( Fig. 1c ) to ease identification of the knot or link formed by the disclination loops ( Fig. 1d ). The variety of states that can be obtained primarily depends on the relative size of the droplet with respect to the chiral pitch, specified in the units of the droplet radius as p 0 =4 R / N . Effectively, the relative chirality parameter N measures the number of π turns of the director along the droplet diameter and does not have to be an integer number. For N ≤3, we only obtain a single disclination loop; however, for N ≥4 the complexity of possible states quickly increases, as a larger number of turns of the cholesteric helix allows stabilization of the disclination lines in a locally trapped state. For N =4, only multiple unlinked loops and Hopf links are obtained, while for N =5, a set of more complex links and knots are found, ranging from symmetric states with one or more isolated loops ( Fig. 2a,b ) to the trefoil knot ( Fig. 1b ), Solomon link ( Fig. 2c ), Hopf link ( Fig. 2d ), Whitehead link ( Fig. 2e ) and a three-component link ( Fig. 2f ), to name a few [39] . Moreover, most of the knots or links are found in many different metastable conformations that differ in the shape and length of the disclinations. Apart from the limited disclination length for a given N , there are no topological restrictions to the knot type, although the more complex knots are seen less frequently. The geometry of the defects affects both the surrounding director field and the energetic stability of the system. The competition of the cholesteric helix with the frustrating effect of the spherical surface forces the disclinations towards the surface of the droplet where they are kept a few nematic correlation lengths away from the surface by the strong surface anchoring. The expulsion of defects is more pronounced when the number of turns per droplet diameter is higher. 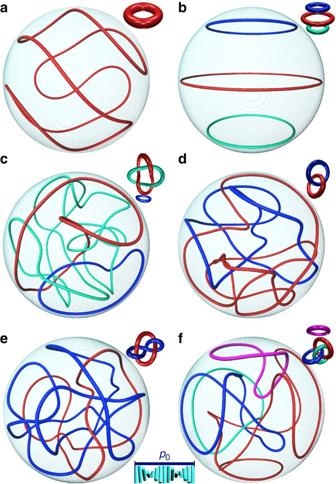Figure 2: Examples of different knots and links as obtained forN=5. (a) A single loop (an unknot), (b) three unlinked loops, (c) Solomon link with an extra loop, (d) a Hopf link, (e) a Whitehead link and (f) a three-component link (633on the Rolfsen table39) with an additional unlinked loop. The disclination lines are drawn as regions of depressed nematic degree of order and colour coded for better visual distinction. The insets show a simplified schematic view of the corresponding knots. The bottom inset shows the pitch and the corresponding cholesteric helix. Figure 2: Examples of different knots and links as obtained for N =5. ( a ) A single loop (an unknot), ( b ) three unlinked loops, ( c ) Solomon link with an extra loop, ( d ) a Hopf link, ( e ) a Whitehead link and ( f ) a three-component link (6 3 3 on the Rolfsen table [39] ) with an additional unlinked loop. The disclination lines are drawn as regions of depressed nematic degree of order and colour coded for better visual distinction. The insets show a simplified schematic view of the corresponding knots. The bottom inset shows the pitch and the corresponding cholesteric helix. Full size image The free energy differences between different states are up to 300 × 10 3 k B T and typically the more symmetric and less knotted structures are more stable. The free energy mainly depends on the length of the disclination line as shown in Fig. 3 , where free energies of various configurations are plotted. The deviation from the linear trend can be attributed primarily to compression of the cholesteric helix caused by frustration, and the difference in the volume of the elastically deformed region around the disclinations in the bulk, compared with the disclinations that run along the boundary. 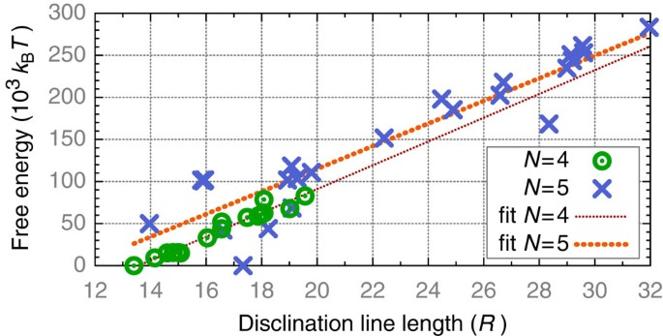Figure 3: Free energy of various metastable states. Free energy, plotted with respect to the measured disclination length, shows a roughly linear dependence. The slopes of the linear regression lines, fit to the calculated data forN=4 and 5, are similar within the margin of data dispersion, at (14,000kBT/R±800kBT/R) and (13,000kBT/R±1,000kBT/R), respectively. The lengths are given in the units of droplet radiusR. Figure 3: Free energy of various metastable states. Free energy, plotted with respect to the measured disclination length, shows a roughly linear dependence. The slopes of the linear regression lines, fit to the calculated data for N =4 and 5, are similar within the margin of data dispersion, at (14,000 k B T / R ±800 k B T / R ) and (13,000 k B T / R ±1,000 k B T / R ), respectively. The lengths are given in the units of droplet radius R . Full size image Linking of disclinations Defects with singularities in the director field can be described in chiral nematics with the same formalism as in achiral nematics. An extended description, in which the helical axis is treated as a separate degree of freedom and also detects defects in the helical order [40] , [41] , is less suitable for our system; as the distortion of layers is large compared with the cholesteric pitch, the helical axis is ill-defined, with extended regions, especially near the surface of the droplet, where twisting is completely suppressed by the restrictive boundary condition. From here on, the only defects we are interested in are singular nematic disclination lines. Topologically stable singular nematic disclinations are characterised by the director field that rotates by π on a path that encircles the disclination. However, there is no topological restriction on the cross-section profile, so the profile behaviour is determined only by the free energy cost and geometric constraints imposed by the confinement. In entangled nematic colloids, the spherical inclusions with homoeotropic anchoring ensure that the director field near the disclination always lies approximately in the plane perpendicular to the disclination tangent. More precisely, the cross-section looks like a 2D nematic defect with a −1/2-winding number, which possesses a characteristic threefold symmetry [18] , [42] . This symmetry can be visualized with a splay-bend parameter ( S SB ; in units of nematic correlation length squared ξ 2 ~44 nm 2 ) that detects varying type of elastic distortion around the disclination [43] . 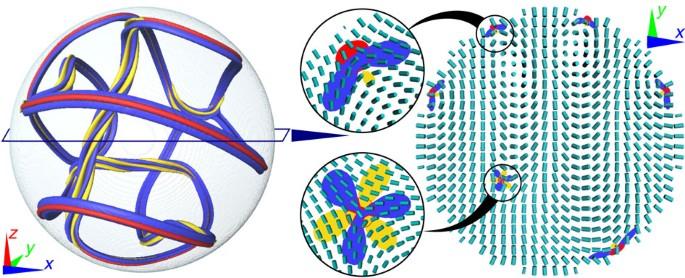Figure 4: Structure of the droplet with a trefoil knot. A nematic disclination line (red isosurface atS=0.48) fromFig. 1b(N=5) with shown regions of higher splay (blue,SSB=0.006) and bend deformations (in yellow,SSB=−0.006) around it. Note the screw-like rotation of the line profile. The director field in a horizontal equatorial section is shown on the right with insets of the line profile near the surface (top inset) and in the bulk (bottom inset). Blue cylinders represent the director field, red regionsS<0.48, while blue and yellow shading marks regions with high splay and bend deformations:SSB>0.006 andSSB<−0.006, respectively. Note the threefold −1/2 profile of the director field surrounding the line that is symmetric in the bulk, becomes distorted near the surface, but not enough to prevent the use of the self-linking number formalism. Figure 4 shows that our system exhibits the same restriction to threefold −1/2-winding number disclinations. In the bulk, the cross-section has no observable deviations from the perpendicular alignment. For the disclinations that lie near the surface of the droplet, the director field tilts out of plane, distorting the threefold cross-section. However, the director field can be always ‘combed’ back to the perpendicular orientation in a continuous manner. The tilting never adds up to topologically significant turning of the director field, but simply fluctuates around the ideal perpendicular orientation. Figure 4: Structure of the droplet with a trefoil knot. A nematic disclination line (red isosurface at S =0.48) from Fig. 1b ( N =5) with shown regions of higher splay (blue, S SB =0.006) and bend deformations (in yellow, S SB =−0.006) around it. Note the screw-like rotation of the line profile. The director field in a horizontal equatorial section is shown on the right with insets of the line profile near the surface (top inset) and in the bulk (bottom inset). Blue cylinders represent the director field, red regions S <0.48, while blue and yellow shading marks regions with high splay and bend deformations: S SB >0.006 and S SB <−0.006, respectively. Note the threefold −1/2 profile of the director field surrounding the line that is symmetric in the bulk, becomes distorted near the surface, but not enough to prevent the use of the self-linking number formalism. Full size image Disclinations from this restricted set, when closed into a loop, possess a topological invariant Sl—self-linking number—that describes a total amount of rotation of the profile around the disclination tangent [42] . This number is quantized in the form Sl= m /3 where loops with an odd m are linked by another disclination, while loops with an even m are not linked. Despite the difference in the elastic-free energy functional, a chiral nematic possesses the same order parameter as the achiral nematic, so the topological discussion of their respective configurations is the same. This means the homotopy theory for nematic defects can be applied. A homoeotropic droplet requires a topological charge q =1 inside, and in a system of disclination loops, the conservation law can be written in terms of the self-linking numbers [42] , Here n is the number of loops, Sl i are the self-linking numbers of individual loops and Lk ij are the linking numbers between pairs of loops. We use a robust algorithm that extracts the ribbons from simulation results to calculate the self-linking numbers without a manual intervention. We take the director field in the neighbourhood of the disclination and use the principle of maximum correlation to track the orientation of the intersection around the loop, measuring the total amount of rotation. Despite deviations from the ideal profile, the assumption that profiles are topologically equivalent to a threefold −1/2 profile is confirmed in all ~150 simulated structures, which include linked and knotted structures consisting of multiple components. Some examples that demonstrate how the conservation (equation (1)) couples topological charge to the linking and self-linking numbers are given in Table 1 . Table 1 Knots with corresponding line length, knot type and Sl number. Full size table Chirality and configuration space The thermal quench simulations show that a large number of different metastable structures can be reached from different random initial conditions. This means that the process of relaxation to the equilibrium state is chaotic and very sensitive to initial conditions, allowing many structures to be reached even without forcing a specific geometry. In most of the resulting structures at least a part of the disclination line resides near the surface of the droplet, which contrasts with the disclination-shortening behaviour in achiral nematics. Here the rewiring of the nematic disclinations is inhibited by layers of π cholesteric twist between the lines. The layers act as barriers, since the unwinding of the helical order is energetically costly, and thus prevent the shortening of the disclinations. These frustration-driven barriers in the free energy are the reason for a large number of metastable states, which only increases with increasing chirality. Despite the fact that the chirality prevents shrinking of the disclinations to a point or a small ring (as would happen in achiral nematics), the free energy is still found to be mainly governed by the disclination length due to its isotropic core ( Fig. 3 ). In contrast to the ordered, lattice-based knots in colloidal systems, which have well-specified rewiring sites [13] , our system has no metric that would allow us to predict the number of different disclination loop conformations. Instead, the space of possible configurations is a continuum. There are no systematic rules to predict and enumerate the structures, so the knots that we observed are but a small fraction of the full set of possibilities. However, the energy landscape continuously depends on the relative chirality parameter N —either by changing the droplet radius or the cholesteric pitch. With the variation of N , the local minima can disappear, merge and move around the configuration space. At N =0, there is only one deep global minimum—the radial hedgehog in the middle. With increasing number of helical turns N , additional local minima with lower symmetry appear and, eventually, the radially symmetric hedgehog state becomes unstable. The nematic braids that we found in droplets at N ~4–6 represent some of the simplest knots and links and conform nicely to the topological rules, derived theoretically for −1/2 disclination loops. With growing N , positions and number of minima in the free energy landscape become practically unpredictable, making the system harder to explore. By further increasing N , we observe not only an increase in the number of metastable states, but also the tendency for the disclination lines to be forced to the layer just below the surface creating structures that are analogous to ones observed in inverted systems—in homoeotropic colloidal particles dispersed in cholesterics [44] . In droplets, the disclinations act as a screening mechanism for the frustrating homoeotropic boundary condition, so that the inside of the droplet can relax to a layer-like structure, locally similar to the cholesteric ground state ( Fig. 5a,b ). When N is sufficiently high, these quasi-2D structures (see also Fig. 5c,d ) become energetically favourable over structures with disclinations passing through the inside of the droplet, which disrupts the layered structure. For N greater than around five turns per diameter, the structures with the lowest energy have the disclinations exclusively restricted to a thin layer right below the surface of the droplet ( Fig. 5 ), although the structures with bulk disclinations still exist as metastable states with much higher free energy. 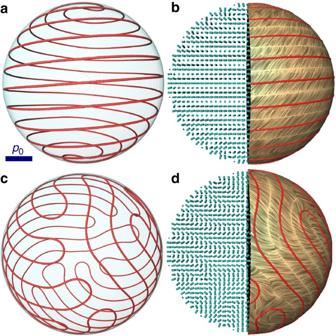Figure 5: Short-pitch droplets with smectic-like subsurface disclinations. (a,b) A stable structure forN=12 with a disclination loop located just below the surface. (b, left) The bulk is filled with a uniformly layered cholesteric director field. (b, right) The director streamlines just below the droplet surface reveal the in-plane component of the director field. (c,d) A metastable state with disclinations in the smectic-like structure and non-uniform cholesteric order in the bulk. Figure 5: Short-pitch droplets with smectic-like subsurface disclinations. ( a , b ) A stable structure for N =12 with a disclination loop located just below the surface. ( b , left) The bulk is filled with a uniformly layered cholesteric director field. ( b , right) The director streamlines just below the droplet surface reveal the in-plane component of the director field. ( c , d ) A metastable state with disclinations in the smectic-like structure and non-uniform cholesteric order in the bulk. Full size image In the limit of cholesterics with high N (note that blue phases are not stable in this regime; see Methods section), the topology of the disclination lines is different from the moderately chiral case. A 2D structure does not allow knots and links but instead exhibits a constant spacing of disclinations, governed by the cholesteric pitch. The resulting surface pattern is similar to a 2D smectic texture, with disclinations acting as smectic layers, and kinks in the disclinations acting as smectic disclinations, which obey topological rules for a smectic on a sphere [45] . Furthermore, the 2D smectic-like disclinations may be interpreted as intersections of bulk cholesteric λ disclinations with the surface. We can estimate the average length of the disclinations in this case as l ~4π R 2 /( p 0 /2)=2π RN , which is a relatively accurate approximation even for the N =4,5 cases (see also Fig. 3 and Table 1 ). The entire range of chirality, from the achiral N =0 to the limit of N →∞, involves an interesting change in topology of the free energy landscape. The topologically rich structures of knots and links that occur around N ~4,5 appear to be a borderline phenomenon at the transition from the single central radial hedgehog at N =0 to the smectic-like pattern of disclinations at the high chirality end of the spectrum. The continuous nature of the chirality parameter opens a question of how the energy minima emerge, evolve, bifurcate and disappear with increasing N . Future research on this problem could reveal hierarchy of metastable states and allow a quantitative exploration of the configuration space continuum. Homoeotropic cholesteric droplets are the first known system that exhibits non-transient knotted singular disclination lines in the bulk. The system has multiple metastable states that persist after relaxation to a local free energy minimum. This allows for observation of relatively complex defect structures present in a simple spherical geometry. Colloidal inclusions are not needed to prevent disclination line rewiring and annihilation. Instead, the intrinsic tendency to form a layered structure is opposed by the spherical confinement enforcing strong but finite homoeotropic anchoring, which creates conditions for topologically non-trivial metastable structures. An increase in topological complexity and potential for knotted structures can be expected not only in droplets but also in other frustrated environments, such as periodic or glass-like microcavities [46] . The presence of bulk disclinations under confinement can also be understood as an intermediate state between the achiral nematic, which tends to a homogenous texture and minimizes the amount of defects as much as topologically allowed, and the blue phases, which contain defects without the need for boundary conditions, and also show non-trivial defect structures when subject to confinement [47] , [48] . The chirality-driven transition from structures with knotted defects in the bulk to structures with all the disclinations residing in the boundary layer close to the surface can be compared with the Meissner effect in superconductors. The role of the penetration depth is played by the cholesteric pitch, and as the surface currents in superconductors screen the unfavourable external magnetic field, the nematic defects screen the frustrating boundary condition, allowing the interior of the droplet to assume the twisted ground state. The spiral surface disclination patterns are similar to those seen around homoeotropic colloidal particles in a cholesteric [14] , except the geometry is inverted. The thermal quench used in our simulations can be reproduced experimentally, by heating the droplet above the isotropic–nematic transition temperature, which means that the knotted structures are feasible in practice. However, if other experimental manipulation techniques are applied, the different parts of the configuration space can be sampled. Changing the initial condition by applying patterned optical beams with varying polarization profile, focal width and intensity, could provide a change in statistics that would allow better control over created knots and links, possibly creating structures unseen in thermal quench simulations. Compared with the organized lattice-based nematic braids in thin nematic cells [13] , [14] , the droplets possess a rotational degeneracy and irregular three-dimensional texture and as such pose harder challenges for experimental manipulation and imaging. Modern observation techniques, such as variants of fluorescence confocal polarizing microscopy [49] , [50] , could be used to probe the three-dimensional structure of the disclinations and compare them with our simulations. The topologically rich occurrence of defects in homoeotropic chiral droplets is an intriguing system to pursue with further refined simulations and to investigate experimentally. As closed systems, the droplets can be observed and manipulated individually, and used in optical experiments as filters, scatterers or resonators. Because of their variety and metastability, the conformation of the droplet could be also used to store information, if reproducible writing and reliable reading could be designed. Further, the diversity of states could be used for marking individual droplets, with the asymmetric texture acting as a marker for tracking translational and rotational motion of the droplets in a flowing medium. Simulation methods To model the chiral LC ordering in homoeotropic cholesteric droplets, a continuum mean field Landau-de Gennes free energy approach is employed [51] . To describe the average orientation and order of the LC molecules, the tensorial order parameter Q ij =( S /2)(3 n i n j − δ ij )+( P /2)( e i (1) e j (1) − e i (2) e j (2) ) is used to construct the total free energy F (where S is the nematic degree of order, n i is the nematic director, P is the biaxiality, e i (1) is the secondary director and e 2 = n × e 1 ). The central interest of this study is the effect of chirality, therefore, we use a single elastic constant approximation of F (ref. 52 ): the LC denotes the integration over the bulk of the LC and D over the surface of the droplet. The first term accounts for the variation of the nematic degree of order S , that is, the possible formation of singular topological defects; A , B and C are material parameters. The elastic distortions from the twisted cholesteric state with a single uniform helical axis, characterized by the pitch p 0 are penalized with the second term with L being the elastic constant in a single constant approximation and q 0 =2π/ p 0 is the inverse pitch. The use of multiple elastic constants (that is, to account for different splay, twist and bend elastic constants) would affect the extent of the areas where the three basic deformation modes were dominant. This would certainly change the free energy and stability of different configurations but would not affect their topological properties and variety of knot types. The final term accounts for the LC interaction with the homoeotropic surface, where W is the anchoring strength and Q ij 0 is the preferred surface orientation (that is, perpendicular to the surface). The homoeotropic anchoring strength W =5 × 10 −3 Jm −2 was chosen as strong but finite and experimentally achievable [53] . The anchoring strength required to keep the disclinations away from the surface linearly depends on the elastic constants and is inversely proportional to the droplet radius, and can be thus much lower for bigger droplets typically used in experiments [54] . The following values for material parameters were used: L =4 × 10 −11 N, A =−0.172 × 10 6 Jm −3 , B =−2.12 × 10 6 Jm −3 , C =1.73 × 10 6 Jm −3 at droplet radius R =1–2.25 μm. The shortest pitch used in our calculations is 0.75 μm, while the blue phases at these material parameters become stable only at twice shorter pitch. We minimize the free energy numerically by using an explicit Euler relaxation finite difference scheme on a cubic grid with typical mesh resolution δ =10 nm to avoid defect pinning. The surface is allocated as a thin spherical shell of mesh points with thickness equal to the mesh resolution. Extraction of disclination geometry We use a custom code to numerically extract the positions and profiles of the disclinations from the simulated data. The position of the disclination line is extracted from the structure and then the nearby director field in a plane perpendicular to the line is compared with the ideal −1/2 disclination profile by calculating the cross-correlation. The maximum of the cross-correlation reveals the best fit of the −1/2 profile to the numerical data. The self-linking numbers are then calculated by using an algorithm proposed by Arai [55] . Once the line is obtained, it can be geometrically simplified to decipher the knot by using the knot relaxation feature in dedicated software KnotPlot. How to cite this article: Seč, D. et al . Topological zoo of free-standing knots in confined chiral nematic fluids. Nat. Commun. 5:3057 doi: 10.1038/ncomms4057 (2014).